A trident dithienylethene-perylenemonoimide dyad with super fluorescence switching speed and ratio Photoswitchable fluorescent diarylethenes are promising in molecular optical memory and photonic devices. However, the performance of current diarylethenes is far from satisfactory because of the scarcity of high-speed switching capability and large fluorescence on-off ratio. Here we report a trident perylenemonoimide dyad modified by triple dithienylethenes whose photochromic fluorescence quenching ratio at the photostationary state exceeds 10,000 and the fluorescence quenching efficiency is close to 100% within seconds of ultraviolet irradiation. The highly sensitive fluorescence on/off switching of the trident dyad enables recyclable fluorescence patterning and all-optical transistors. The prototype optical device based on the trident dyad enables the optical switching of incident light and conversion from incident light wavelength to transmitted light wavelength, which is all-optically controlled, reversible and wavelength-convertible. In addition, the trident dyad-staining block copolymer vesicles are observed via optical nanoimaging with a sub-100 nm resolution, portending a potential prospect of the dithienylethene dyad in super-resolution imaging. During the past several decades, intensive investigation has been devoted to photochromic materials because of their potential applications ranging from rewritable data storage [1] and optical switching [2] to chemical sensing [3] . The development of novel molecular photoswitches is attributed to organic synthetic chemists, whereas in the past decade more interests have been focused on the application of current popular molecular photoswitches such as 1,2-dithienylethene (DTE) [4] , [5] , [6] . The photoisomerization reactions of DTE derivatives are reversible upon light irradiation but thermally irreversible, which are appealing for molecular optical memory and optical switches in photonic devices [4] . The ultraviolet–visible absorption spectroscopy is usually used for tracking the change of colour (photochromism) by monitoring the absorbance of DTEs at maximum absorption wavelength. Alternatively, fluorescent spectroscopy exhibiting high sensitivity provides another method to characterize the photoswitching properties of DTEs, which requires those DTEs that display both photochromism and fluorescence switching. Evidently, fluorescence switching is more promising than photochromism in all-optical switches and transistors [7] , [8] , [9] . A great deal of efforts have been taken to develop novel photoswitchable fluorescent DTE derivatives with high fluorescence quantum yields ( Φ F ), on/off ratios and switching speeds [10] , [11] , [12] , [13] , [14] , [15] , [16] . However, the performance of photoswitchable fluorescent DTEs is far from satisfactory owing to the scarcity of high-speed switching capability and large fluorescence on/off ratio. Especially, the fluorescence quenching ratios of DTEs at the photostationary state (PSS) are not paid as much attention as that of DTEs at isolated closed form [17] . Generally, for a fluorescent DTE, part of the open form would be converted to closed form and reach its PSS after ultraviolet irradiation. As a result, the fluorescence would be quenched partly at the PSS because there are still unconverted open-form DTEs, which contribute to the remnant fluorescence. To minimize the remnant fluorescence at the PSS, multiple DTEs linked on one fluorophore have been proposed. In the pioneering investigation of Irie’s group [18] in 2001, they designed a compound containing two DTE moieties electronically conjugated with a bis(phenylethynyl)-anthracene residue. The Φ F of its isolated closed form is low to 0.001, but the conversion efficiency and the fluorescence quenching of DTE at the PSS are no more than 25%. The DTE electronically conjugated with fluorophore may weaken the photochromic capability of DTE and thus quenching ratio and photochromic sensitivity. Tian et al . [19] reported on fluorescent tetraazaporphyrins-fused quadruple-DTEs, in which the cyclization of the DTEs units at the two counter-positions occurs at the same time. The Φ F of open form is lower than 10% but no detail about closed form is given. The cyclization speed seems slow because it takes a long time (45 min) to reach its PSS after ultraviolet irradiation. It is observed again in their reported another compound in which two DTEs are attached to perylene-diimide [20] . 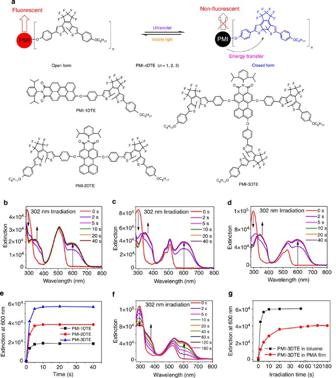Figure 1: Absorption properties of PMI-nDTEs. (a) The schematic photochromism and fluorescence photoswitching of perylenemonoimide (PMI) modified by three diethienylethenes (DTEs): PMI-1DTE, PMI-2DTE and PMI-3DTE. (b–d) Time-dependent ultraviolet–visible spectra of PMI-1DTE (b), PMI-2DTE (c) and PMI-3DTE (d) in toluene and their optical density change at 600 nm (e) upon 302-nm ultraviolet irradiation. The concentration is 1.0 × 10−6M. (f) Time-dependent ultraviolet–visible spectra of PMI-3DTE in polymethylacrylate (PMA) film upon 302 nm irradiation. (g) Optical density changes at 600 nm of PMI-3DTE in toluene and PMA film with time upon 302-nm ultraviolet irradiation. It does not mean that the fluorophores substituted with multiple DTEs would definitely show fast photochromic speed and high-fluorescence quenching ratio according to the previously reported results ( Supplementary Table 1 ). No matter how great the fluorescence quenching property of isolated DTE, it is impossible to isolate the closed form from the materials because the DTEs are used in situ in optoelectronic devices. Hence, the fluorescence switching properties of DTEs at the PSS should be the determined factor for practical optical application and we need to address in situ fluorescence quenching speed and quenching ratio of fluorescent DTEs at the PSS. In terms of molecular design, we should consider not only the individual properties of DTE and the fluorophore but also the electron interaction between functional groups when we seek for improving the photochromic sensitivity of DTE and accomplishing the high-contrary fluorescence between the bright (open-form) and dark (PSS) state of photoswitchable fluorophores. With the above in mind, we have proposed that multiple DTEs are linked with perylenemonoimide (PMI) through an oxygen bridge. In recent years, PMIs have been extensively investigated because of their excellent photostability, high-fluorescence quantum yields both in solution and solid state [21] , [22] . Combining stable photoswitching of DTE and bright fluorescence of PMI would help endow fluorescence photoswitching behaviour with high-speed switching capability and large fluorescence on/off ratio [23] . Here we have designed and synthesized a series of photoswitchable fluorophores PMI- n DTE ( n =1, 2, 3), where n is the number of DTEs linked on single PMI subunit via covalent coupling of oxygen bridge. PMI is a typical fluorophore having high Φ F and photostability, whereas three DTE units together in one PMI-3DTE molecule act as much more efficient photochromic fluorescent resonance energy transfer activators than a single DTE unit. In this work, the quantitative relations between fluorescence quenching efficiencies, cyclization yields and ultraviolet irradiation time in dilute solution are deduced theoretically and confirmed experimentally. The photochromic fluorescence quenching ratio of PMI-3DTE in the PSS exceeds 10,000 and fluorescence quenching efficiency is close to 100% in seconds of ultraviolet irradiation. The prototype optical device based on PMI-3DTE enables the optical switching of incident light and conversion from incident light wavelength to transmitted light wavelength, indicating that PMI-3DTE-based optical device is all-optically controlled, reversible and wavelength-convertible. The PMI-3DTE-staining block copolymer vesicles are observed via optical nanoimaging with sub-100 nm resolution. Design and synthesis of PMI- n DTE The photochromism and fluorescence switching of PMI- n DTEs ( n =1, 2, 3) and their molecular structures are shown in Fig. 1a . Fluorescent PMI and one, two and three photochromic DTE units are covalently linked through oxygen spacers affording PMI modified by one, two and three DTE units, namely PMI-1DTE, PMI-2DTE and PMI-3DTE, respectively. The detailed synthesis and characterization are provided in Supplementary Methods and Supplementary Fig. 1 . Figure 1: Absorption properties of PMI- n DTEs. ( a ) The schematic photochromism and fluorescence photoswitching of perylenemonoimide (PMI) modified by three diethienylethenes (DTEs): PMI-1DTE, PMI-2DTE and PMI-3DTE. ( b – d ) Time-dependent ultraviolet–visible spectra of PMI-1DTE ( b ), PMI-2DTE ( c ) and PMI-3DTE ( d ) in toluene and their optical density change at 600 nm ( e ) upon 302-nm ultraviolet irradiation. The concentration is 1.0 × 10 −6 M. ( f ) Time-dependent ultraviolet–visible spectra of PMI-3DTE in polymethylacrylate (PMA) film upon 302 nm irradiation. ( g ) Optical density changes at 600 nm of PMI-3DTE in toluene and PMA film with time upon 302-nm ultraviolet irradiation. 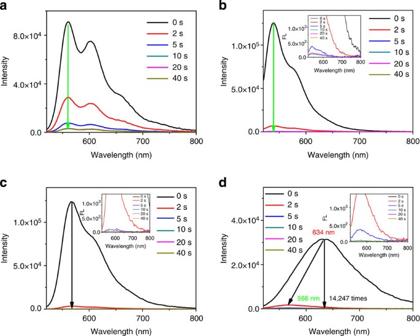Figure 2: Emission properties of PMI-nDTEs. Fluorescence spectral changes of PMI-1DTE (a), PMI-2DTE (b), PMI-3DTE (c) in toluene upon irradiation with 302-nm light. (d) Fluorescence intensity changes of PMI-3DTE in PMA film (PMI-3DTE/PMA=2.4:100 (w/w)) upon irradiation with 302 nm. The concentration is 1.0 × 10-6M. The excitation wavelength is 514 nm. Full size image Photochromism The optical properties of PMI- n DTEs have been investigated and summarized in Table 1 and Supplementary Table 2 . Figure 1 shows the absorption spectra of PMI- n DTEs upon irradiation with 302-nm light in solution and in polymethylacrylate (PMA) film. The electronic spectra of PMI- n DTE display an intense absorption band at 500–530 nm with a molar extinction coefficient more than 30,000 l mol −1 cm −1 ( Table 1 ), which is assigned to the PMI subunit ( Supplementary Figs 2–6 ). PMI- n DTEs undergo conspicuous photochromic reactions in solution upon irradiation with 302-nm light for 2–5 s. The absorption band in the red region ( λ max =600 nm) is assigned to the closed form of DTE. The molecular extinction coefficients of open-form PMI- n DTEs at λ max (~300 nm) are as high as 4.0 n × 10 4 l mol −1 cm −1 , and those of the closed form at ~600 nm are about 1.9 n × 10 4 l mol −1 cm −1 ( Table 1 ). The molar extinction coefficient of PMI-3DTE at 600 nm is almost three times of that of PMI-1DTE, whereas PMI-2DTE is twice of that of PMI-1DTE ( Fig. 1b–e ). However, for three PMI- n DTEs, the times to attain the PSS are scarcely different ( Fig. 1e ). Compared with organic solvents, their photochromic speed in polymer film becomes much slower. It takes about 50 s to attain 90% of the absorbance at PSS of PMI-3DTE in PMA film ( Fig. 1f ). In addition, it is difficult to attain high conversion from open- to closed-form. The photocyclization conversion of PMI-3DTE in PMA is only about 70% of that in toluene ( Fig. 1g ). Table 1 Optical properties of PMI-1DTE, PMI-2DTE and PMI-3DTE in toluene. 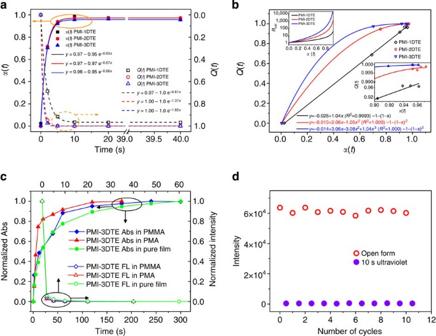Figure 3: Photokinetics and fluorescence switching. (a) Photoconversion yieldsα(t) and fluorescence quenching efficiencyQ(t) monoexponentially change with timet.α(t) was fitted well withy=1−ekx, whereasQ(t) fitted well withy=1−enkx, wherekis the rate constant,nis the number of DTEs in one PMI-nDTE. (b) The polynomial fitting of fluorescence quenching efficiencyQ(t) versus photoconversion yieldα(t). The inset at right side: zooms inb. The inset at top left corner is the calculated fluorescence quenching ratioRcal=1/[1−α(t)]n. The concentration is 1.0 × 10−6M in toluene. (c) Absorbance (600 nm) and fluorescence intensity (maximum emission wavelength) changes of PMI-3DTEs in PMMA, PMA and pure films under 302-nm irradiation time. (d) Reversible fluorescence switching for PMI-3DTE in pure film at 634 nm upon alternating irradiation with 302-nm (10 s) and visible light greater than 495 nm (5 min). The excitation wavelength for fluorescence is 514 nm. Full size table Upon 302-nm ultraviolet irradiation, the open-form DTEs in PMI- n DTEs are converted to the closed form DTEs with a yield above 95% ( Table 1 and Supplementary Table 3 ) at PSS in toluene. 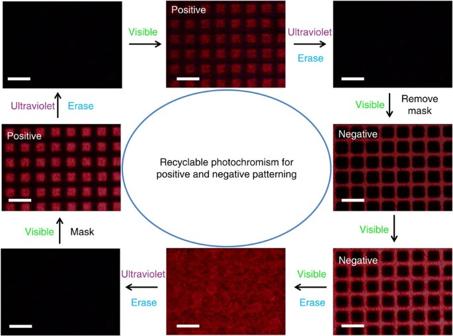Figure 4: Photo-rewritable fluorescence patterning. The PMA flim doped with PMI-3DTE (PMI-3DTE/PMA=2.4:100 (w/w)) is spin-coated on the surface of an glass slide. A copper mask is put on the film or moved away during the experiment. The fluorescence of the film is observed on a fluorescence microscope under a green light excitation by alternating irradiation of ultraviolet (302 nm, hand-held lamp, 0.8 mW cm−2) and visible light (>495 nm). Scale bar, 50 μm. The photocyclization quantum yields Φ o→c of PMI- n DTEs were measured according to the literature method [24] , [25] ( Supplementary Note 1 and Supplementary Table 4 ): Φ o→c (PMI-1DTE)=0.425±0.008, Φ o→c (PMI-2DTE)=0.497±0.009, Φ o→c (PMI-3DTE)=0.495±0.009, respectively. Usually, the Φ o→c for most of DTEs would not exceed 0.5 owing to the 1:1 proportion of parallel and anti-parallel conformation [19] . Therefore, the DTE in PMI- n DTEs system shows competitive ultraviolet sensitivity and contributes to the excellent fluorescence photoswitching performance. The cycloreversion quantum yields Φ c→o at 617-nm irradiation were determined 0.008±0.0002, 0.007±0.0002, 0.007±0.0001 for PMI-1DTE, PMI-2DTE and PMI-3DTE, respectively. Fluorescence properties of open-form PMI- n DTEs Figure 2 and Supplementary Figs 2–5 show the fluorescence spectral change of PMI-DTEs along with the photocyclization. The initial Φ F of PMI-1DTE, PMI-2DTE and PMI-3DTE in toluene is 85%, ~100% and 97%, respectively ( Table 1 ). The photoluminescence (PL) spectra of PMI- n DTEs exhibit a red shift of emission wavelength and a decrease of Φ F when the solvent polarity increases. This is because that photoinduced electron transfer in donor–acceptor structure happens in polar solvent, here phenoxy group as a donor and PMI as an acceptor. Compared with other two compounds, PMI-2DTE without a DTE at peri -position shows much weaker fluorescence in polar solvent and more sensitive to polarity ( Supplementary Fig. 6 ). It is interesting that the emission wavelengths of PMI-1DTE and PMI-3DTE in toluene are almost the same, whereas PMI-2DTE shows >30 nm blue shift ( Table 1 ). Compared with PMI, all the PMI- n DTEs have DTEs attached to a perylene core via phenoxy groups, which are of electron-donating ability. From the density functional theory (DFT) calculation, the electron cloud density of the peri -position phenoxy group is more than that of bay -position ( Supplementary Fig. 7 ). Those peri -position phenoxy groups increase the π-conjugation of the whole system more than that of bay -position. That is the reason why all three PMI- n DTEs show red-shift fluorescence compared with that of PMI ( Supplementary Fig. 8 ). Reasonably, PMI-3DTE with three DTEs possesses the largest emission peaks at 567 nm. However, PMI-2DTE lacks a DTE at peri -position of PMI compared with PMI-1DTE and PMI-3DTE, but possesses two DTEs at its bay -positions. From the DFT calculation, the twist angles of PMI core are ~0°, 16.35° and 15.26° for PMI- n DTE ( n =1, 2, 3), respectively ( Supplementary Fig. 7 ). The DTEs at the bay -positions cause the planar perylene core twisted. Accordingly, the DTE at peri -position increases more efficiently the π-conjugation than two DTEs at bay -position. Therefore, the emission peak of PMI-2DTE (539 nm) shows blue shift compared with that of PMI-1DTE (561 nm), whereas only a little red shift relative to that of PMI (531 nm). For the same reason, PMI-1DTE without two bay -position DTEs shows slightly blue shift fluorescence relative to PMI-3DTE (567 nm). Figure 2: Emission properties of PMI-nDTEs. Fluorescence spectral changes of PMI-1DTE ( a ), PMI-2DTE ( b ), PMI-3DTE ( c ) in toluene upon irradiation with 302-nm light. ( d ) Fluorescence intensity changes of PMI-3DTE in PMA film (PMI-3DTE/PMA=2.4:100 (w/w)) upon irradiation with 302 nm. The concentration is 1.0 × 10 -6 M. The excitation wavelength is 514 nm. Full size image Photoswitchable fluorescence The fluorescence intensity promptly decreases and is quenched almost completely upon 2–5 s of 302-nm ultraviolet irradiation. In comparison, the fluorescence quenching of PMI-1DTE and PMI-2DTE becomes much slower than that of PMI-3DTE ( Fig. 2a–c ). Even in PMA medium, PMI-3DTE fluorescence is almost quenched in 2 s ( Fig. 2d ). Upon irradiation with visible light >495 nm, the fluorescence gradually returns to the initial intensity again. The fluorescence on/off switching ratio increases from PMI-1DTE, PMI-2DTE to PMI-3DTE ( Supplementary Table 2 ). The fluorescence on/off switching ratio of PMI-1DTE at PSS in toluene is 30. For PMI-2DTE in toluene, the value at PSS becomes 865, much better than PMI-1DTE. For PMI-3DTE, the fluorescence on/off switching ratio at PSS in toluene becomes 3,026. The fluorescence on/off switching ratio of PMI-3DTE at PSS in polymethyl methacrylate (PMMA) film is 1,634, whereas the value in PMA film even attains 14,247, an unprecedented fluorescence quenching value, which indicates that the fluorescence (FL) on/off ratio is matrix dependent ( Supplementary Fig. 9 ). The results are encouraging and competent in the application environments requiring super switching speed and high-fluorescence on/off switching ratio [26] , [27] , [28] . In addition, the photodynamic processes of PMI- n DTEs monitored by absorption and fluorescence spectra have been investigated in dilute toluene solution. For all PMI- n DTEs, 5 s of ultraviolet irradiation time is enough to attain their 90% PSS ( Supplementary Table 2 ). The photoconversion yields of cyclization α ( t ) of PMI- n DTEs are quite approximate at any time and independent on the number of DTEs attached to one PMI fluorophore ( Supplementary Note 2 ). Upon the ultraviolet irradiation, the α ( t ) of PMI- n DTEs increase monoexponentially with time t and the fitting results approximate α ( t )=1− e kt with very high coefficients of determination R 2 >0.999 ( Fig. 3a ), in which k is the rate constant and determined by the intensity of ultraviolet light absorbed by each kind of DTE on PMI- n DTEs ( Fig. 3a ). It indicates that the photoisomerization reactions of PMI- n DTEs under those conditions employ a first-order kinetics [1− α ( t )]=1 × e kt . The speeds for photochromism (colour change) under 302-nm ultraviolet irradiation are similar and do not depend on how many DTEs attached to PMI in dilute solutions. Figure 3: Photokinetics and fluorescence switching. ( a ) Photoconversion yields α ( t ) and fluorescence quenching efficiency Q ( t ) monoexponentially change with time t . α ( t ) was fitted well with y =1− e kx , whereas Q ( t ) fitted well with y =1− e nkx , where k is the rate constant, n is the number of DTEs in one PMI- n DTE. ( b ) The polynomial fitting of fluorescence quenching efficiency Q ( t ) versus photoconversion yield α ( t ). The inset at right side: zooms in b . The inset at top left corner is the calculated fluorescence quenching ratio R cal =1/[1− α ( t )] n . The concentration is 1.0 × 10 −6 M in toluene. ( c ) Absorbance (600 nm) and fluorescence intensity (maximum emission wavelength) changes of PMI-3DTEs in PMMA, PMA and pure films under 302-nm irradiation time. ( d ) Reversible fluorescence switching for PMI-3DTE in pure film at 634 nm upon alternating irradiation with 302-nm (10 s) and visible light greater than 495 nm (5 min). The excitation wavelength for fluorescence is 514 nm. Full size image However, for fluorescence switching, the situation is different. After 2 s of ultraviolet irradiation, the fluorescence quenching efficiencies of PMI- n DTEs are 69.6%, 94.6% and 97.3%, respectively ( Fig. 3a ), showing ultra-fast fluorescence quenching speed for PMI-3DTE. Although the fluorescence changes of PMI-2DTE and PMI-3DTE are much ahead of that of the absorption, the fluorescence quenching efficiencies Q ( t ) should be dependent on the photoconversion yields α ( t ). For PMI- n DTEs system, the emission spectra of PMI overlap significantly with the absorption spectra of the closed form of the DTE subunit. Moreover, PMI is covalently linked DTE through oxygen bridge with a quite small distance. Thus, the intramolecular energy transfer efficiency from PMI to closed-form DTE would be extremely high [24] and is measured experimentally almost 100% ( Supplementary Note 3 ) [17] , [23] . In single PMI- n DTE molecule, one closed-form DTE is presumed to be enough to quench the fluorescence of PMI completely. The fact is that the photocyclization reaction cannot be completed usually in single DTE (the yields are ~97% for PMI- n DTEs). If the open form cannot be converted to closed form completely, there is always fluorescence from remained open form unless we can separate out the non-fluorescent isolated closed form. For the dilute solution of PMI-1DTE, the quenching efficiency Q ( t ) depends on the proportion of closed form α ( t ), Q ( t )=1−[1− α ( t )]. Both of them change with time t . Sequentially, the fluorescence quenching on/off ratio R ( t )=1/[1− α ( t )]. The fluorescence quenching speed keeps pace with photochromism process for PMI-1DTE. If multiple DTEs are integrated with one PMI to get PMI-2DTE and PMI-3DTE, the probability of all the DTEs in one molecule keep open form decreases sharply after ultraviolet irradiation, namely, [1− α ( t )] n . Thus, Q ( t )=1−[1− α ( t )] n and R (t)=1/[1− α ( t )] n . The more the DTEs, the lower the probability of all the DTEs in open form at the same time and the more sensitive the fluorescence quenching upon ultraviolet irradiation. Experimentally, for PMI-1DTE, there is only single DTE linked to PMI. After 302-nm ultraviolet irradiation, PMI-1DTE attains its PSS with photoconversion 96.2% calculated by 1 H-NMR. There is 3.8% open form remaining in PSS of DTE and the calculated fluorescence on/off value is about 26. That is why the measured fluorescence on/off ratio of PMI-1DTE is only about 30. In comparison, the conversion yield of PMI-2DTE at PSS after 302-nm irradiation is 97.2% calculated by NMR. The proportion of both DTEs at open form in one PMI-2DTE molecule is 0.0787% and the calculated fluorescence on/off value is about 1,270, which is closed to the value 865 measured from PL spectrum. This is also applicable for PMI-3DTE. The conversion yield of PMI-3DTE at PSS is 95.4% calculated by 1 H-NMR. The proportion of all three DTEs at open form in one PMI-3DTE molecule is 0.0095% and the correspondingly fluorescence on/off value is calculated about 10,500, which is reasonable compared with the value 3,026 measured from PL spectrum. The difference between the quenching ratio measured from PL spectrum and calculated from 1 H-NMR for PMI-3DTE may be related to the background of solvents and the baseline of the PL equipment. The weak fluorescence of PMI-3DTE at PSS is nearly out of the limitation of detection ( Supplementary Fig. 6 ). The polynomial function fitted curve of the measured quenching efficiency Q ( t ) versus conversion α ( t ) for PMI-1DTE in toluene is nearly linear, y =−0.026+1.04 x ≈ x =1−(1− x ), whereas those for PMI-2DTE and PMI-3DTE are y =−0.01+2.06 x −1.05 x 2 ≈ x 2 −2 x =1−(1− x ) 2 and y =−0.014+3.06 x −3.08 x 2 +1.04 x 3 ≈− x 3 +3 x 2 + x =1−(1− x ) 3 , respectively, with very high coefficients of determination R 2 >0.999 ( Fig. 3b ). On the whole, the experimental data conform very well with the theoretical polynomial function y =1−(1− x ) n , that is, Q ( t )=1−[1− α ( t )] n . As a result, the fluorescence quenching ratio of PMI-3DTE in dilute solution is much larger than that of PMI-2DTE and PMI-1DTE ( Fig. 3b ) at the same conversion yield. As α ( t )=1− e kt has been described above, it is deduced that Q ( t )=1− e nkt , which overlaps significantly the corresponding fitting curves y =1− e nkx ( Fig. 3a ). Accordingly, the conversions α ( t ) of PMI- n DTE in dilute solution should be the same at any time t , whereas the number of DTEs is the main fact dramatically affecting fluorescence switching speed and ratio. PMI-3DTE shows different behaviours in photoswitching speed, fluorescent intensity and their on/off ratio depending on the surrounding matrices ( Fig. 3c ). In solid film, the conformational transition of PMI-3DTE molecule is significantly restricted by the surrounding matrix. Therefore, the photochromic process in solid film becomes more difficult than that in solution. Moreover, in pure PMI-3DTE film, the molecular conformational transition is restricted more seriously due to the smaller free volume of PMI-3DTE molecules than in PMMA and PMA film. It takes more than 300 s to reach its PSS in pure film, whereas only 120–180 s for PMMA and PMA film. In PMMA film with a glass transition temperature ( T g ) at 104 °C, the absorption band of PMI-3DTE at 600 nm increases slowly upon 302 nm irradiation, 10 s to attain less 50% PSS, whereas 10 s to attain 75% PSS in PMA films ( T g =~0 °C). This result demonstrates that the photochromic (colour change) speed is lower in PMMA film with higher T g . It is surprising that the fluorescence quenching speed of PMI-3DTE in solid film is comparable to that in solution. It takes only 2 s of ultraviolet irradiation to quench 96–98% of the fluorescence of PMI-3DTE in PMA, PMMA and pure films and after 10 s, the fluorescence of PMI-3DTE is quenched more than 99.2% ( Table 2 ). Therefore, the fluorescence quenching of PMI-3DTE in solid state is much more efficient than photochromism of PMI-3DTE. In dilute solution, only intramolecular energy transfer usually exists. However, the intermolecular energy transfer [29] from light emitting molecules to the surrounding closed-form DTE molecules contributes significantly to the fluorescence quenching because of the much larger molecular packing density in solid film, especially in pure film with a huge quenching ratio closed to ∞ ( Supplementary Table 2 ). In PMA film, the emission peak is about 634 nm, which is similar to solid film (640 nm), whereas it is 580 nm for PMMA film. It is reasonable that the PMI-3DTE molecules aggregate compactly in pure film, resulting in large red shift emission at 640 nm. The large difference in emission wavelength in PMA and PMMA films indicates that the PMI-3DTEs molecules are inclined to aggregate in PMA film with much lower T g than PMMA film probably because of the relatively poor miscibility between nonpolar PMI-3DTE and polar PMA matrix. That is why PMI-3DTE in PMA film could keep both fast photochromic speed and high-fluorescence quenching ratio above 10 4 . The excellent fluorescence switching properties of PMI-3DTE in solid film enable PMI-3DTE to be used as an inspiring material in optical applications. Table 2 Fluorescence quenching efficiencies of PMI-3DTE in solid films upon 302-nm irradiation. Full size table The reversibility of the fluorescence switching process can be demonstrated by cycling forward and backward, between the open- to closed-form. When PMI-3DTE in PMMA solid film is excited at 514 nm, the strong emission at 584 nm in the beginning and above 99% fluorescence quenching after ultraviolet irradiation for 10 s are monitored ( Supplementary Fig. 9 ). PMI-3DTE shows certain fatigue resistance after photoannealing for ten ultraviolet–visible irradiation cycles. Comparably, pure PMI-3DTE film shows decent reversibility and better fatigue resistance in cycling behaviour at alternating ultraviolet and visible light irradiation ( Fig. 3d and Supplementary Fig. 10 ). Photo-rewritable fluorescence patterning Photo-rewritable fluorescence patterning on PMI-3DTE in polymer film is investigated by structured illumination through Cu-grid photomask ( Fig. 4 ). The periodic pattern of Cu grid with emissive square array is recorded as a positive image, which is subsequently erased by 302-nm ultraviolet light. The negative patterning image with structured grid-like fluorescence was recorded upon visible excitation after removing Cu grid, which is then erased by visible light in minutes. The photochromism and fluorescence switching upon alternating ultraviolet–visible illumination can be recycled to develop and erase different positive and negative patterns by the aid of photomask. This successful demonstration of erasable fluorescence imaging on the polymer film enables instantaneous application of PMI-3DTE as one kind of photoink for rewritable printing, ultrahigh-density rewritable optical memory media or imaging processes. Figure 4: Photo-rewritable fluorescence patterning. The PMA flim doped with PMI-3DTE (PMI-3DTE/PMA=2.4:100 (w/w)) is spin-coated on the surface of an glass slide. A copper mask is put on the film or moved away during the experiment. The fluorescence of the film is observed on a fluorescence microscope under a green light excitation by alternating irradiation of ultraviolet (302 nm, hand-held lamp, 0.8 mW cm −2 ) and visible light (>495 nm). Scale bar, 50 μm. Full size image All-optical transistors The photons as information carriers are comprehensively investigated and promising in information technology with demands on bandwidth and information density [8] , [9] . Organic molecular switches may provide potential capability to applications in transmit, modulate and detect light or photons. Previous investigation of DTE derivatives indicates extreme potentials as all-optical transistors, whereas the fluorescence on/off ratio is not very high [7] . Here we attempt to demonstrate the potential of PMI-3DTE with the highest fluorescence on/off ratio and switching speed as a prototype of all-optical transistor. 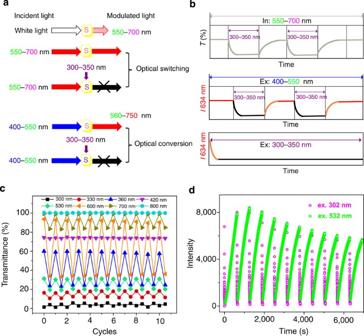Figure 5: All-optical switch and transistor. (a) Schematic of the optical switching, wavelength conversion and modulation. Ex: excitation wavelength;T(%): transmittance. (b) Time-domain description of incident light irradiations or excitations and corresponding optical response of the molecule. (c) Transmittance recorded at 300, 330, 360, 420, 530, 600, 700 and 800 nm at subsequent ultraviolet–visible illumination cycles. (d) Fluorescence switching of subsequent switching cycles at alternating 302- and 532-nm excitation. PMI-3DTE in PMA film (PMI-3DTE/PMA=2.4:100 (w/w)). Excitation wavelength: 302 and 532 nm. Emission wavelength: 634 nm. Figure 5 shows the schematic illumination and experimental results of the optical switching, wavelength conversion and modulation. Figure 5: All-optical switch and transistor. ( a ) Schematic of the optical switching, wavelength conversion and modulation. Ex: excitation wavelength; T (%): transmittance. ( b ) Time-domain description of incident light irradiations or excitations and corresponding optical response of the molecule. ( c ) Transmittance recorded at 300, 330, 360, 420, 530, 600, 700 and 800 nm at subsequent ultraviolet–visible illumination cycles. ( d ) Fluorescence switching of subsequent switching cycles at alternating 302- and 532-nm excitation. PMI-3DTE in PMA film (PMI-3DTE/PMA=2.4:100 (w/w)). Excitation wavelength: 302 and 532 nm. Emission wavelength: 634 nm. Full size image The film of open-from PMI-3DTE retains high transmittance of visible light above 550 nm, whereas the closed form shows a broad absorption band at around 480–700 nm blocking the transmission of corresponding light. Open-form PMI-3DTE emits red fluorescence upon visible excitation (400–550 nm), which means that the incidental blue or green light is transformed to red output light (560–750 nm). However, after exposed to 300–350-nm ultraviolet light, the object become a ‘black hole’, which absorbs all light throughout visible region and thus no output visible light can be observed. Thus, all-optical modulation integrating switching and conversion is enabled to be accomplished in single optical device based on PMI-3DTE organic molecular photoswitch ( Fig. 5a ). A solution of 2.4 mg PMI-3DTE and 100 mg PMA in 50 ml tetrahydrofuran (THF) was prepared and then coated on the quartz substrate. The optical density and emission intensity were monitored upon ultraviolet–visible light excitation. Figure 5d shows the transmittance switching of PMI-3DTE film at eight selective wavelengths ranging from 300 to 800 nm. As shown in Fig. 1f , PMI-3DTE in solid film exhibits the minimal absorption difference at 330, 420, 530, 700 and 800 nm before and after ultraviolet irradiation, whereas the peaks at 360 and 600 nm change significantly. The transmittance at 420 nm preserves constant upon alternating ultraviolet–visible illumination. The photochromic PMI-3DTE can effectively switch the transmission of light at 360 and 600 nm upon alternative ultraviolet and visible light irradiation, whereas it is not efficient for other wavelengths such as 300, 330 and 530 and 800 nm. The results indicate that PMI-3DTE accomplishes an all-optically tuned, recyclable and wavelength-selective optical switching. As shown in Fig. 2d , PMI-3DTE in solid film exhibits the divergent difference of emission intensity at 634 nm resulting from PMI. The irradiations with 302 and 532 nm induce the positive ring-closed and reverse ring-open isomerization of PMI-3DTE. Also PMI-3DTE can launch red emission upon the excitation with 302 and 532 nm light. Thereby, we could monitor the change of emission intensity at 634 nm upon 302 and 532 nm excitation. Figure 5d shows the fluorescent switching of PMI-3DTE film upon alternating ultraviolet (302 nm) and visible light (532 nm) excitation. The emission intensity of PMI-3DTE film decreases promptly upon 302 nm of excitation because of the photocyclization of open-form PMI-3DTE. Subsequently, switching the excitation from 302 to 532 nm triggers the reverse cycloreversion of closed-form PMI-3DTE, resulting in the fluorescence increase at 634 nm. The wavelength conversion from input green light (532 nm) to output red light (634 nm) can be reversibly tuned by ultraviolet light (302 nm). The result in Fig. 5 indicates the optical device based on fluorescence switching of PMI-3DTE is all-optically controlled, reversible and wavelength convertible. Optical nanoimaging Multiphase nanostructures from self-assembly of block copolymers are promising in nanolithography and nanostructure templating. The goal of visualizing the nanoscopic domains has stimulated numerous investigations on imaging methods, including scanning electronic microscopy, transmission electronic microscopy, atomic force microscopy and scanning tunnel microscopy. However, these methods are invasive, high-vacuum or time-consuming so that their application is limited. For optical microscopy, the diffraction of light limits the spatial resolution of conventional fluorescence microscopy with about 200–300 nm in the lateral direction and 500–700 nm in the axial direction. In the past decades, some novel optical nanoimaging named as super-resolution fluorescence microscopy techniques have been developed to exceed the diffraction barrier by the sequential localization of individual fluorescent molecules, such as stochastic optical reconstruction microscopy [30] and photoactivated localization microscopy [31] . These methods have achieved an order of magnitude enhancement in spatial resolution down to 20 nm over conventional fluorescence microscopy. Here we design a proof-of-concept system by staining the vesicles in water formed from block copolymer polystyrene- b -poly-(ethylene oxide) (PSt- b -PEO, PSt Mn38000, PEO Mn11000) using photoswitchable PMI-3DTE probe. The photoswitching properties of PMI-3DTE with super fluorescence switching speed and on/off ratio enable sub-diffraction optical nanoimaging of block copolymer nanostructures. It is observed that PSt- b -PEO block copolymer vesicles in bright-field image ( Fig. 6a ) are comparable with the transmission electron microscopic and scanning electronic microscopic images in shapes and sizes ( Fig. 6a inset and Supplementary Fig. 11 ). The on and off fluorescence of PMI-3DTE can be cycled under exposure to continuous 302-nm ultraviolet light (~0.40 mW cm −2 ) and intermittent 405-nm laser (~10 mW cm −2 ; Fig. 6c,d ), in which the 405-nm light only excites the fluorophore causing emission at 634 nm. The merged image from bright-field and fluorescence imaging is shown in Fig. 6b . PSt- b -PEO block copolymer was self-assembled with PMI-3DTE staining and observed by our home-built photoswitching nanoimaging system followed by algorithm processing [32] . Based on the discussion of fluorescence microscopy above, it is confident that most fluorescence of PMI-3DTE displayed in the fluorescence images in Fig. 6b is located in the hydrophobic double layer of block copolymer vesicles because of the higher emissive and hydrophobic nature of PMI-3DTE. Evidently, for the fluorescent pattern within the hydrophobic double layers of block copolymer vesicles, most of the fluorescent bilayers are so close that sub-diffraction nanostructures become indistinguishable in conventional fluorescent images ( Fig. 6c ). On the contrary, photoswitching nanoimaging in Fig. 6e,f clearly demonstrates nanoscale localization of emissive PMI-3DTE staining agents in the hydrophobic bilayers of block polymer vesicles affording basic contour of polymer vesicles. For example, The full-width at half-maximum of the localized single fluorescent point in Fig. 6g (zoom in from Fig. 6f ) is determined from Gaussian deconvolution as low as to 36 nm ( Fig. 6h ). Meanwhile, two fluorescent points of 62 nm apart can be well differentiated in the photoswitching nanoimaging ( Fig. 6i,j ). Thus, the photoswitching nanoimaging method is capable of high localization precision down to 36 nm, which is comparable to that of scanning electron microscopy imaging of organic materials. 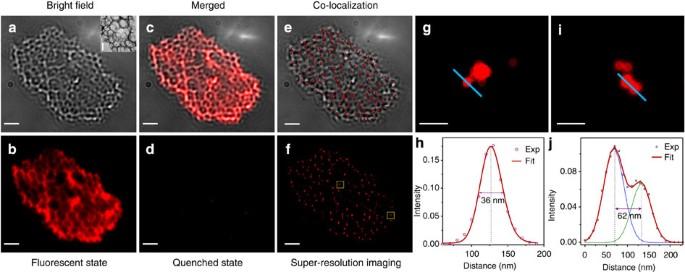Figure 6: Optical nanoimaging. (a) Bright-field image of block copolymer polystyrene-b-poly-(ethylene oxide) (PSt-b-PEO) vesicles stained with PMI-3DTE, inset: transmission electronic microscopy image; scale bar, 1 μm; (b) fluorescence image; (c) merged image; (d) fluorescence image at quenched state; (e) photoswitching nanoimaging co-localization with bright image; (f) photoswitching nanoimaging; (g,i) expanded view of the marked regions inf. Fluorescence cross-sectional profiles of single fluorescent point (h) and a pair of vicinal fluorescent points (j) along the dashed lines ingandi, respectively. Scale bar ofa–f, 2 μm. Scale bar ofgandi, 200 nm. Figure 6: Optical nanoimaging. ( a ) Bright-field image of block copolymer polystyrene- b -poly-(ethylene oxide) (PSt- b -PEO) vesicles stained with PMI-3DTE, inset: transmission electronic microscopy image; scale bar, 1 μm; ( b ) fluorescence image; ( c ) merged image; ( d ) fluorescence image at quenched state; ( e ) photoswitching nanoimaging co-localization with bright image; ( f ) photoswitching nanoimaging; ( g , i ) expanded view of the marked regions in f . Fluorescence cross-sectional profiles of single fluorescent point ( h ) and a pair of vicinal fluorescent points ( j ) along the dashed lines in g and i , respectively. Scale bar of a – f , 2 μm. Scale bar of g and i , 200 nm. Full size image People usually consider photochromism when molecular photoswitches are paid attention. Researchers have attempted adjusting the fluorescence of one or two fluorophores by using single DTE, whereas the fluorescence quenching ratio and speed are limited by the cyclization yield. Several works refer to the structure that single fluorophore is connected by conjugated coupling with two or more DTEs, whereas the fluorescence cannot be quenched efficiently, possibly owing to complicated electronic conjugation or energetic interaction of molecular components. In order to figure out the effects of DTEs on the fluorescence of fluorophore, we design and synthesize a series of PMI-nDTE ( n =1, 2, 3) with non-conjugated oxygen-bridge linkage between PMI and multiple DTEs, which keeps the properties of two components relatively independent. The short distance of each closed-form DTE and PMI in PMI-3DTE ensures almost 100% of energy transfer efficiency, whereas the multiple independent DTEs increase the quenching speed and ratio exponentially. In this scheme, the photochromic speed has not changed, which only depends on DTEs from the point of mechanism, whereas the switching speed of fluorescence increases greatly. High fluorescence quantum yield of PMI and higher molar ratio of DTE/PMI groups in PMI-3DTE result in bright emission of open form along with higher fluorescence on/off ratio. That matches incredibly the requirements of high performance of DTE derivatives in their applications. Especially, the almost dark state can be obtained for PMI-3DTE. That benefits the high noise-signal ratio and low-threshold readout when applying DTE in optical memory, reversible fluorescence patterning and all-optical transistors and so on. In addition, the result of PMI-3DTE in optical nanoimaging provides a potential photoswitchable fluorophore for super-resolution imaging. In conclusion, we report on a new molecular design principle of a trident PMI modified by three DTEs having high fluorescence switching speed and so-far-highest fluorescence on/off ratio. The fluorescence is reversibly quenched based on photochromic fluorescent resonance energy transfer from PMI to DTE units when the DTE units convert between the open- and the closed-ring isomers upon irradiation with visible and ultraviolet light. The photochromic fluorescence quenching ratio of PMI-3DTE in PSS exceeds 10,000 and fluorescence quenching efficiency is closed to 100% in seconds of ultraviolet irradiation. The transmittance and emission switching experiments on the prototype device based on PMI-3DTE have been designed and conducted. From the optical switching of transmittance and emission of PMI-3DTE in solid film devices, all-optical transmittance switching at selective wavelengths and wavelength conversion of visible light frequency is demonstrated. The simultaneous accomplishment of all-optical modulation in light intensity and wavelength enables the promising application of PMI-3DTE devices in all-optical systems of visible light frequency. The photoswitching nanoimaging demonstrates that block copolymer vesicles could be imaged with higher resolution than that obtained by conventional fluorescent imaging. The unique molecular design of PMI-3DTE provides prospective opportunity of fluorescent molecular switches in optical devices and super-resolution imaging. Materials All solvents, reagents and chemicals are commercially available and used as supplied, unless otherwise stated. Chloroform is dried over calcium hydride with stirring overnight followed by distillation under reduced pressure. THF is dried using sodium wire-benzophenone system and distillation. Dimethoxyethane is bubbled with N 2 for 30 min before use. N -Bromosuccinimide is recrystallized from water. The preparation and characterization of PMI-1DTE, PMI-2DTE and the precursors of PMI- n DTE are reported in detail in Supplementary Methods and Supplementary Figs 12 and 13 . PMI-3DTE is synthesized following below procedures. N -(2,6-Diisopropylphenyl)-1,6,9-tris(4-bromophenoxyl)-perylene-3,4-dicarboximide ( 8 ) Compound 7 (0.36 g, 0.50 mmol), 4-bromophenol (0.35 g, 2.0 mmol) and potassium carbonate (0.21 g, 2.0 mmol) were stirred in N-methyl-2-pyrrolidone (NMP) (20 ml) at 130 °C for 4 h. After cooling down to room temperature, the reaction mixture was poured into hydrochloric acid aqueous (1.0 M, 200 ml). The resulting precipitate was washed with water and dried. The crude product was purified by column chromatography on silica gel using 50% dichloromethane in hexane as eluent, and the first fraction was collected to get 0.20 g red solid with a yield of 40%. 1 H NMR (600 MHz, CDCl 3 ): δ 9.31 (d, J =7.8 Hz, 1H), 9.13 (d, J =8.8 Hz, 1H), 8.42 (d, J =8.2 Hz, 1H), 8.32 (s, 1H), 8.29 (s, 1H), 7.64 (t, J =8.1 Hz, 1H), 7.53 (d, J =8.8 Hz, 2H), 7.50–7.43 (m, 5H), 7.30 (d, J =7.8 Hz, 2H), 7.04 (d, J =8.8 Hz, 2H), 7.02 (d, J =8.8H, 2 Hz), 6.95 (t, J =6.0 Hz, 2H), 6.90 (d, J =8.8 Hz, 1H), 2.70 (dq, J 1 =13.6, J 2 =6.8 Hz, 2H), 1.14 (d J =6.8 Hz, 12H,); 13 C NMR (151 MHz, CDCl3): δ 162.9, 155.4, 155.2, 155.1, 155.04, 152.4, 151.7, 145.6, 133.2, 133.2, 133.2, 131.6, 130.6, 130.5, 129.8, 129.8, 129.6, 128.2, 128.1, 127.4, 126.4, 126.0, 125.6, 125.5, 124.5, 124.3, 124.0, 122.4, 122.0, 121.9, 121.1, 120.0, 119.9, 117.38, 116.7, 116.6, 112.3, 29.1, 24.0; matrix-assisted laser desorption/ionization–time of flight–mass spectrometry ( m / z ): [M+1] + calcd. for C 52 H 36 Br 3 NO 5 , 993.0132; found, 994.078; HPLC purity: 99.5%, eluting with DCM: hexane=3: 7. N -(2,6-Diisopropylphenyl)-1,6,9-tris[4-(4,4,5,5-tetramethyl-[1,3,2]dioxaborolan-2-yl)-phenyl]-perylene-3,4-dicarboximide ( 9 ) Compound 8 (0.20 g, 0.20 mmol) and bis(pinacolato)diboron (0.31 g, 1.20 mmol) were mixed together with potassium acetate (0.15 g, 1.50 mmol) in dioxane (20 ml) under a light stream of nitrogen. Finally, PdCl 2 (dppf) catalyst (22 mg, 0.030 mmol) was added, and the reaction mixture was stirred under nitrogen atmosphere for 16 h at 90 °C. After cooling down, the reaction mixture was extracted with DCM, washed with water three times, dried over with MgSO 4 , concentrated under reduced pressure. The crude product was chromatographed on silica gel eluting with DCM/hexane 8:2 and recrystallized in DCM/hexane binary solvents to yield a red solid (0.12 g, 54%). 1 H NMR (400 MHz, CDCl 3 ): δ 9.33 (d, J =7.8 Hz, 1H), 9.15 (d, J =8.8 Hz, 1H), 8.38 (d, J =8.2 Hz, 1H), 8.33 (s, 1H), 8.31 (s, 1H), 7.83 (t, J =8.9 Hz, 4H), 7.79 (d, J =8.5 Hz, 2H), 7.59 (t, J =8.1 Hz, 1H), 7.43 (t, J =7.8 Hz, 1H), 7.28 (d, J =7.8 Hz, 2H), 7.16–7.08 (m, 4H), 7.05 (d, J =8.5 Hz, 2H), 6.92 (d, J =8.8 Hz, 1H), 2.71 (dq, J 1 =13.7, J 2 =6.8 Hz, 2H), 1.39–1.31 (m, 33H), 1.14 (d, J =6.8 Hz, 12H); 13 C NMR (151 MHz, CDCl 3 ): δ 163.0, 159.0, 158.7, 155.2, 152.3, 151.5, 145.7, 137.1, 137.1, 136.9, 131.7, 130.7, 129.8, 129.8, 129.4, 128.5, 128.4, 127.5, 126.8, 126.2, 126.1, 126.0, 124.5, 124.4, 124.0, 122.5, 121.8, 121.0, 119.1, 117.4, 117.2, 113.1, 83.9, 83.9, 83.8, 29.1, 24.9, 24.0; high-resolution mass (atmospheric pressure chemical ionization) ( m / z ): [M+1] + calcd. for C 70 H 72 B 3 NO 11 , 1,135.5385; found, 1,136.5454. PMI-3DTE (13) To a 10-ml two-neck round flask, compound 4 (0.39 g, 0.65 mmol), compound 9 (0.11 g, 0.11 mmol), Na 2 CO 3 (0.17 g, 1.62 mmol), water (2.5 ml) and dimethoxyethane (10 ml) were added under N 2 atmosphere, then the catalyst Pd(PPh 3 ) 4 (19 mg, 0.016 mmol) was added under N 2 stream. The reaction mixture was refluxed at 90 °C for 24 h. After cooling down, water (50 ml) and ethyl ether (50 ml) were added and the organic layer was washed with water (50 ml × 3), dried over Na 2 SO 4 and concentrated under reduced pressure. The crude product was purified by gravity silica-gel column chromatography (silica gel) eluting with hexane DCM/hexane (3:2) to yield a red solid (0.090 g, 37%). 1 H NMR (600 MHz, CDCl 3 ): δ 9.39 (d, J =7.7 Hz, 1H), 9.20 (d, J =8.8 Hz, 1H), 8.46 (d, J =8.2 Hz, 1H), 8.37 (s, 1H), 8.34 (s, 1H), 7.67 (t, J =8.1 Hz, 1H), 7.58 (d, J =8.6 Hz, 2H), 7.55 (d, J =8.7 Hz, 2H), 7.52 (d, J =8.7 Hz, 2H), 7.48–7.39 (m, 7H), 7.30 (d, J =7.8 Hz, 2H), 7.27-7.25 (overlap with CDCl 3 , 2H), 7.21 (d, J =11.1 Hz, 2H), 7.18 - 7.14 (m, 6H), 7.09 (d, J =8.7 Hz, 2H), 6.97 (d, J =8.8 Hz, 1H), 6.92–6.87 (m, 6H), 4.00–3.92 (m, 6H), 2.72 (dt, J 1 =13.6, J 1 = 6.8 Hz, 2H), 2.04–1.85 (m, 18H), 1.81–1.75 (m, 6H), 1.50–1.40 (m, 6H), 1.38–1.27 (m, 24H), 1.18–1.10 (m, 12H), 0.89 (t, J =6.8 Hz, 9H); 13 C NMR (151 MHz, CDCl 3 ): δ 163.1, 159.1, 159.1, 155.8, 155.6, 155.5, 152.6, 151.9, 145.6, 142.4, 142.3, 141.3, 141.2, 140.3, 140.1, 131.7, 130.7, 130.6, 130.0, 129.8, 129.8, 129.6, 129.5, 129.5, 129.4, 128.2, 128.1, 127.6, 127.6, 127.5, 127.4, 126.9, 126.1, 126.0, 126.0, 125.9, 125.9, 125.9, 125.7, 125.7, 125.6, 125.4, 124.5, 124.2, 124.0, 122.5, 122.4, 122.3, 122.3, 121.9, 121.1, 121.1, 121.0, 120.6, 120.4, 118.9, 118.8, 115.0, 114.5, 112.5, 67.9, 31.8, 29.4, 29.3, 29.2, 29.1, 26.1, 26.0, 24.0, 22.7, 14.6, 14.1; matrix-assisted laser desorption/ionization–time of flight–mass spectrometry ( m / z ): 2,467.473 [M] + ; high-resolution mass (atmospheric pressure chemical ionization) ( m / z ): [M+1] + calcd. for C 139 H 123 F 18 NO 8 S 6 , 2,467.7286; found, 2,468.7324; HPLC purity: 99.1%, eluting with DCM/hexane=2:8. Optical properties measurement The ultraviolet–visible spectrum was recorded using a Shimadzu ultraviolet–visible-NIR Spectrophotometer (UV-3600). The PL spectrum was recorded using Edinburgh instruments (FLS920 spectrometers). For the measurement of the fluorescence time profiles, time-correlated single-photon counting method using a picosecond pulsed light emitting diode (EPLED-445, 442.8 nm, Pulse width=95.3 ps, the Instrument response function is 44.5 ps) with 8 MHz repetition rate was employed. The 302 nm ultraviolet (2.67 mW cm −2 ) irradiation for the ‘ring-closing’ reaction was performed using an ultraviolet transmission platform, and the visible light for the ‘ring-opening’ reaction was obtained from a common household table lamp (25 W) and a long-wavelength pass filter (495 nm, Accessories of FLS920 spectrometer). The 617-nm visible light was from a Red-Orange (617 nm) LUXEON Rebel LED (2.28 mW cm −2 , Lumileds Lighting). For the cyclization/cycloreversion quantum yields measurement, a quartz cuvette with black wall was used while it is a fluorescence quartz cuvette for other optical test. For the demonstration of all-optical transistor, a solution of 2.4 mg PMI-3DTE and 100 mg PMA in 50 ml THF was prepared and then coated on the quartz substrate. The absorption and fluorescent spectra were recorded and the optical density and emission intensity were monitored upon ultraviolet–visible light excitation. In all-optical transistor experiment, the fluorescence intensity at 302 nm/532 nm excitation was adjusted to be the same order of magnitude by changing slit value. Conventional fluorescence microscopy and photoswitching nanoimaging Amphiphilic block copolymer PSt- b -PEO (molecular weight: PSt 38000, PEO 11000) vesicles were used for encapsulation of hydrophobic photoswichable fluorescent diarylethene molecules. The block copolymer vesicles were prepared by interfacial instabilities of emulsion droplets method [32] . Chloroform solutions containing 10 mg cm −3 PSt- b -PEO and 0.2 mg cm −3 PMI-3DTE were prepared first and then mixed with 1 mg cm −3 SDS aqueous solution. After that, the obtained mixture was shaken vigorously to get organic solvent-in-water emulsion. As chloroform was volatilized slowly into air, the emulsion droplets were shrinking. The organic solvent/water interface became unstable and spontaneously formed a new interface, finally resulting in dispersion of the copolymer as vesicular aggregates wrapping PMI-3DTE in the aqueous solution. The obtained vesicles were dispersed on a ultra-clean glass slide with drop-coating method. The morphologies of vesicles were characterized on a photoswitching imaging optical setup, which was based on a home-built microscope setup consisting of an Olympus IX 71 inverted optical microscope, a × 100/numerical aperture=1.49 oil immersion TIRF objective (UAPON 100XOTIRF, Olympus), 473 nm solid-state laser (CNILaser), a 302-nm ultraviolet lamp and a sCMOS camera (Flash2.8, Hamamatsu). During photoswitching nanoimaging, electronic shutters (UNIBLITZ VS14, Vincent Associates) were used to control the duration of laser irradiance, and a dichroic mirror (FF509-FDi01, Semrock) and a long pass filter (BLP01-561R-25, Semrock) were used to separate the collected fluorescence from scattering laser and impurity fluorescence. We used an Image J plugins written in Java by ourselves to analyse the image [33] . The movies were collected at a frame rate of ~50 Hz and all durations were 5,000 frames. When the fluorescence of polymer was quenched during the imaging after 302-nm ultraviolet irradiation, a weak 473-nm laser was flashed to recover the density. We then repeated this cycle many times to get enough images for further photoswitching nanoimage reconstruction. How to cite this article : Li, C. et al . A trident dithienylethene-perylenemonoimide dyad with super fluorescence switching speed and ratio. Nat. Commun. 5:5709 doi: 10.1038/ncomms6709 (2014).